Above-room-temperature ferroelectricity and antiferroelectricity in benzimidazoles The imidazole unit is chemically stable and ubiquitous in biological systems; its proton donor and acceptor moieties easily bind molecules into a dipolar chain. Here we demonstrate that chains of these amphoteric molecules can often be bistable in electric polarity and electrically switchable, even in the crystalline state, through proton tautomerization. Polarization–electric field ( P–E ) hysteresis experiments reveal a high electric polarization ranging from 5 to 10 μC cm −2 at room temperature. Of these molecules, 2-methylbenzimidazole allows ferroelectric switching in two dimensions due to its pseudo-tetragonal crystal symmetry. The ferroelectricity is also thermally robust up to 400 K, as is that of 5,6-dichloro-2-methylbenzimidazole (up to ~373 K). In contrast, three other benzimidazoles exhibit double P–E hysteresis curves characteristic of antiferroelectricity. The diversity of imidazole substituents is likely to stimulate a systematic exploration of various structure–property relationships and domain engineering in the quest for lead- and rare-metal-free ferroelectric devices. Ferroelectricity, that is, electric polarity in solids or liquid crystals that is switchable with the electric field E , is in increasing demand as it provides diverse entries into electronic, electromechanical, optical and optoelectronic applications [1] , [2] , [3] . In ferroelectrics, the spontaneous electric polarization P at E =0 can be reversibly inverted by reversing the electric field, and the polarization–electric field ( P–E ) curve then shows a hysteresis loop. The related antiferroelectricity phenomenon exhibits a double P–E hysteresis curve when the dipolar arrangement is reversed stepwise through the antipolar arrangement at low electric field [4] . A very high polarization response, which is promising for capacitors, memories and piezoelectric applications, has so far been discovered mostly in inorganic oxides containing toxic lead or rare elements, such as bismuth, tantalum, niobium and so on. The high-performance piezoelectricity of lead-based ceramics is often related to competing ferroelectric and antiferroelectric orders [3] , [5] . To decrease our reliance on these materials and to work towards a green and sustainable society, purely organic ferroelectrics [6] , [7] , which are expected to be used as key materials in organic, printable and bendable electronic device applications, are being pursued as possible alternatives. Recent advances in piezoresponse force microscopy (PFM) have also revealed the nanoscale ferroelectricity of crystalline γ-form glycine and porcine aortic walls [8] , [9] . Here we demonstrate that imidazoles carrying large electric dipoles constitute a new family of single-component ferroelectrics, as well as antiferroelectrics, in the bulk state with variable chemical substituents. In an earlier supramolecular approach using acid and base molecules, proton donor and acceptor moieties were joined together to host the proton dynamics for switching the bistable polarities [8] . This principle was recently extended to single-component compounds; the proton tautomerism on O−H…O bonds achieves excellent room-temperature ferroelectricity in croconic acid [7] , β-diketone enols and carboxylic acids [10] . There are, however, some drawbacks specific to each compound for the fabrication of thin-film devices. For instance, croconic acid is corrosive and also requires a strong acid for crystallization. Some O−H…O-bonded organic ferroelectrics are unstable against air oxidation, whereas others are thermally fragile. Satisfying all the performance and process-compatibility demands together with sufficient electric, mechanical and environmental endurance is a challenging task. The imidazole ring is an important building block in biological systems, as exemplified by histidine, histamine and vitamin B 12 ( [11] , [12] , [13] ). In addition, these compounds are now currently utilized as ingredients in various ionic liquids [14] , as well as a corrosion inhibitor for copper. Many derivatives are commercially available, stable in air and highly soluble in alcohols and other common organic solvents. The small imidazole molecule carries a large dipole moment (3.61 D) directed nearly parallel to the N−H bond. Imidazole can both donate and accept protons with modest acidity [15] , and this amphoteric nature has been exploited as a guest proton carrier in porous coordination polymers designed for anhydrous proton-conductive materials working at high temperatures [16] . In the crystalline state, the chemical mechanism designated in Fig. 1a is anticipated for the polarization reversal. Unless the substituents allow for steric hindrance or distinct hydrogen bonding, imidazole moieties can spontaneously assemble into a linear chain structure because of the directional nature [17] of the intermolecular N−H…N bonds. The polarity of the chain can be inverted cooperatively by the concomitant π-bond switching and proton transfer that alters the N−H…N bond to N…H−N and vice versa. It should be noted that the scheme shown in Fig. 1a is generalized for various combinations of substituents X, Y 1 and Y 2 . Therefore, the discovery of above-room-temperature ferroelectricity and antiferroelectricity that we report here will stimulate a systematic exploration of various structure–property relationships in the quest for lead- and rare-metal-free ferroelectric devices. 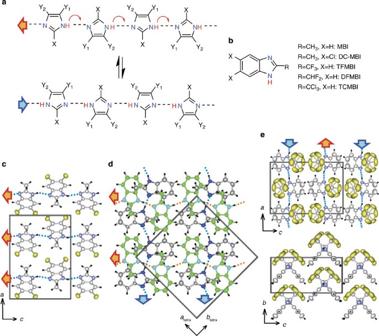Figure 1: Chemical and crystal structures of ferroelectric and antiferroelectric imidazoles. (a) Hydrogen bonding (broken lines) and polarization reversal mechanism through the proton tautomerism of the imidazole moiety. (b) Chemical structures of the ferroelectric and antiferroelectric benzimidazoles. Abbreviations are given for the imidazole derivatives. (c) Ferroelectric DC-MBI crystal viewed along the crystallographicbdirection. (d) Pseudo-tetragonal molecular arrangement and hydrogen-bonded sequences therein of the ferroelectric MBI. (e) Molecular arrangement of the antiferroelectric TCMBI crystal viewed along the crystallographicb(top) andadirections (bottom). The CCl3group is in rotational disorder over two conformations. Figure 1: Chemical and crystal structures of ferroelectric and antiferroelectric imidazoles. ( a ) Hydrogen bonding (broken lines) and polarization reversal mechanism through the proton tautomerism of the imidazole moiety. ( b ) Chemical structures of the ferroelectric and antiferroelectric benzimidazoles. Abbreviations are given for the imidazole derivatives. ( c ) Ferroelectric DC-MBI crystal viewed along the crystallographic b direction. ( d ) Pseudo-tetragonal molecular arrangement and hydrogen-bonded sequences therein of the ferroelectric MBI. ( e ) Molecular arrangement of the antiferroelectric TCMBI crystal viewed along the crystallographic b (top) and a directions (bottom). The CCl 3 group is in rotational disorder over two conformations. Full size image Structural assessment To scrutinize these chemical schemes, we focused first on the imidazoles of Y 1 =Y 2 and their ring-fused analogues, benzimidazoles ( Fig. 1b ), because a number of related compounds have already been deposited in the Cambridge Structural Database. We searched the database for linear chain structures having some pseudo-symmetry to determine which candidate ferroelectrics have so far been overlooked, but we did not encounter this example in the literature. The 5,6-dichloro-2-methylbenzimidazole (DC-MBI) crystal belongs to the orthorhombic system with the space group Pca 2 1 (no. 29). The polarity of all the hydrogen-bonded chains was found to align along the crystal c direction ( Fig. 1c ). The global structure can be satisfactorily refined with slightly higher R factors under the higher crystal symmetry of Pbcm (no. 57) by locating a mirror symmetry plane normal to the molecular plane. In this model, the protons inevitably occupy disordered or centred locations between two nitrogen atoms. The alternative approach is to determine the disordered or centred location of the protons. If this crystal structure represents the paraelectric state, then the protons may be ordered as asymmetric N−H…N bonds form at temperatures lower than the Curie point and host ferroelectricity or antiferroelectricity. The other possibility is the artefacts arising from a pseudo-symmetry element assumed in the analysis misled by the global structure of minute deviation from the higher symmetry. We found that this occurs in the 2-methylbenzimidazole (MBI) crystal. The reported MBI crystal structure [18] belongs to the tetragonal system with the symmetric space group P 4 2 / n (no. 86). The protons are disordered over two sites, and their hydrogen bonds form straight bands running along either [110] tetra or the crystallographically equivalent [1[macr1]0] tetra direction. In our analysis, the tetragonal lattice is barely lowered to the monoclinic system with the space group Pn (no. 7), which is one of the maximal subgroups of P 4 2 / n by interchanging the crystallographic b and c axes. Because the as-grown MBI crystals ( Supplementary Fig. S1 and Supplementary Table S1 ) are not in a single-domain state but easily mix the tetragonal a and b axes, the axes and plane indices are presented here according to the tetragonal symmetry. The proton ordering is responsible for the polarity within the (001) tetra plane in the bulk ( Fig. 1d ). Ferroelectric properties We measured the P–E hysteresis curves for both the MBI and DC-MBI crystals with the applied electric field parallel to the hydrogen-bonded molecular sequence direction: E ||[110] tetra for MBI and E ||[001] for DC-MBI. At room temperature, the MBI crystal exhibited ferroelectricity with quasi-rectangular loops and a remanent polarization as large as 5.2 μC cm −2 ( Fig. 2a ). The coercive field determined from the P =0 intercept is 11 kV cm −1 at 0.2 Hz and increases with frequency. Symmetry breaking from the tetragonal lattice permits polarization switching with any electric field direction parallel to the (001) tetra plane. In fact, measurements with electric field configurations of E ||[100] tetra and orthogonal E ||[010] tetra applied separately to two pieces cut from the same single crystal confirmed the apparent isotropic value of the remanent polarization within the (001) tetra sheet (3.9–4.0 μC cm −2 , see Supplementary Fig. S3a and Supplementary Discussion ). The ferroelectricity was also confirmed at higher temperatures of up to 400 K from the P–E hysteresis loops, which exhibited little change in the remanent polarization but did exhibit a decrease in the coercive field with temperature ( Fig. 2b and Supplementary Fig. S3b ). 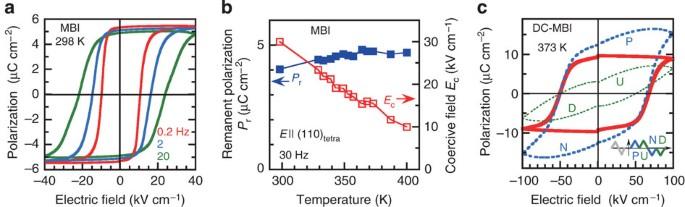Figure 2: Ferroelectric properties. (a) Electric polarization (P) versus electric field (E) hysteresis loops of [110]tetrapolarization in MBI measured at room temperature with a triangular ac electric field of various frequencies (f=0.2–20 Hz). (b) Temperature dependence of the remanent polarization and coercive field of MBI obtained from the [110]tetrahysteresis loops withf=30 Hz. (c) The dielectric hysteresis of thec-direction polarization in DC-MBI atT=373 K measured using the double-wave method with a triangular ac electric field off=5 Hz (see inset for schematic of applied waveform). The pure hysteresis component (solid curve) was obtained by subtracting the ‘non-hysteresis’ polarization (up (U) and down (D) runs) from the total (positive (P) and negative (N) runs). Figure 2: Ferroelectric properties. ( a ) Electric polarization ( P ) versus electric field ( E ) hysteresis loops of [110] tetra polarization in MBI measured at room temperature with a triangular ac electric field of various frequencies ( f =0.2–20 Hz). ( b ) Temperature dependence of the remanent polarization and coercive field of MBI obtained from the [110] tetra hysteresis loops with f =30 Hz. ( c ) The dielectric hysteresis of the c -direction polarization in DC-MBI at T =373 K measured using the double-wave method with a triangular ac electric field of f =5 Hz (see inset for schematic of applied waveform). The pure hysteresis component (solid curve) was obtained by subtracting the ‘non-hysteresis’ polarization (up (U) and down (D) runs) from the total (positive (P) and negative (N) runs). Full size image The DC-MBI crystal exhibited a coercive field at room temperature that was too high to complete a satisfactory loop even with the maximum field of 100 kV cm −1 . The hard switching likely reflects the elevated potential barrier for a proton to hop between the bistable potential minima because of the elongated N…N distance (2.98 Å) compared with that of MBI (2.91 Å on average). The spontaneous polarization was evaluated by reducing the coercive field at elevated temperatures. A hysteresis curve could be discerned at temperatures >300 K. Additional contributions from electrical conduction (leakage) through the sample were suggested by the longitudinally warped P–E curves of the raw data, but this warping could be eliminated by the double-wave method [19] by applying a double-triangular waveform voltage (see inset in Fig. 2c for the applied waveform). The quasi-parallelogram of the hysteresis contribution thus extracted from the data at 373 K gave a large remanent polarization of 10 μC cm −2 and coercive field of about 60 kV cm −1 ( Fig. 2c ). Ferroelectric domain structure The pseudo-tetragonal symmetry of MBI allows the relative orientation of the polarization in perpendicular (90°) configurations as well as conventional antiparallel (180°) configurations. To verify the multi-domain structure in the single crystal composed of both 90° and 180° domains, we employed PFM (Methods). The topography ( Fig. 3a ) of the cleaved (001) tetra surface shows a step-and-terrace profile with a step height of, predominantly, c /2 or c (~7.2 Å), reflecting the layered structure of MBI. The corresponding in-plane piezoresponse image is shown in Fig. 3b , where four kinds of ferroelectric domains are clearly discerned. A sequence of PFM measurements with a distinct cantilever geometry (see Supplementary Fig. S6 ) enabled us to identify the directions of the local polarizations P local , which were determined to be along any [100], [−100], [010] or [0–10] direction in the pseudo-tetragonal setting. This then demonstrates the existence of 90° domain walls in terms of PFM, which is consistent with the apparent isotropic remanent polarization mentioned above. We note that the pattern of the observed domain configurations is richer than our original expectation; the prevailing 90° domain walls often merge at a single point to form vortex and anti-vortex structures. Similar vortex structures have recently been reported in BiFeO 3 thin films [20] , where the vortices are artificially created, or written, by scanning the cantilever with dc bias. 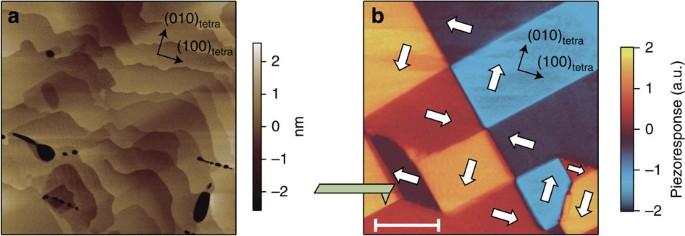Figure 3: PFM image of MBI single crystal. (a) Topography image of the cleaved [001]tetrasurface. (b) In-plane piezoresponse image. The geometry of the cantilever is illustrated schematically, and the directions of the local polarizations are indicated by white arrows. The scale bar corresponds to 4 μm. Figure 3: PFM image of MBI single crystal. ( a ) Topography image of the cleaved [001] tetra surface. ( b ) In-plane piezoresponse image. The geometry of the cantilever is illustrated schematically, and the directions of the local polarizations are indicated by white arrows. The scale bar corresponds to 4 μm. Full size image Antiferroelectric properties The polarization was reversed at room temperature by applying an electric field parallel to the hydrogen-bonded chain for the other three imidazoles: 2-trifluoromethylbenzimidazole (TFMBI), 2-difluoromethylbenzimidazole (DFMBI) and 2-trichloromethylbenzimidazole (TCMBI) (see Fig. 1b ), and their P–E curves, as shown in Fig. 4 , are similar. At low electric fields, the polarization increases linearly with E , whereas quasi-step-like changes appear at higher fields with hysteresis. This double hysteresis loop is characteristic of antiferroelectricity, which appears when the free energy of an antipolar arrangement of dipolar chains is comparable to that of a polar arrangement. By subtracting the normal dielectric (linear P–E ) component, we obtained electrically induced polarizations of about 8, 6 and 8 μC cm −2 for TFMBI, DFMBI and TCMBI, respectively. Such large polarizations are comparable to the remanent polarization of DC-MBI, signalling the fully aligned polarity of the dipolar chains under an electric field beyond the critical field. 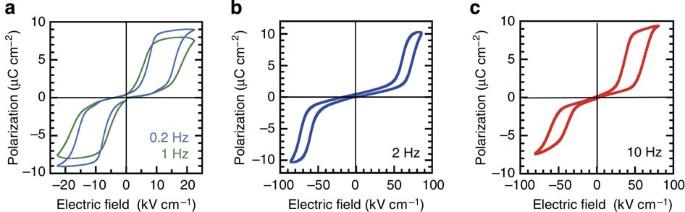Figure 4: Antiferroelectric properties at room temperature. The applied electric field was parallel to the direction of the hydrogen-bonded molecular sequence. (a) TFMBI, (b) DFMBI and (c) TCMBI crystals. Molecule abbreviations are given inFig. 1b. Figure 4: Antiferroelectric properties at room temperature. The applied electric field was parallel to the direction of the hydrogen-bonded molecular sequence. ( a ) TFMBI, ( b ) DFMBI and ( c ) TCMBI crystals. Molecule abbreviations are given in Fig. 1b . Full size image According to our crystal structural analysis, these antiferroelectrics have similar molecular and hydrogen-bonded chain structures ( Supplementary Fig. S5 ). It should be noted that the large thermal ellipsoid over two sites for each halogen atom corresponds to the rotational disorder of the trihalomethyl groups in the TFMBI and TCMBI crystals. By ignoring the proton locations, these antiferroelectric molecules have pseudo-mirror symmetry normal to the molecular plane. In reality, both the molecular and crystal symmetries are lowered by the proton ordering. The three-dimensional molecular arrangements of these crystals are not isomorphous to one another. Although ferroelectricity requires a polar crystal structure, antiferroelectricity is usually related to the nonpolar structure at E =0, which is true for the TFMBI and DFMBI crystals, as they exhibit an antipolar arrangement of dipolar chains. Because of the proton ordering, the pseudo-orthorhombic lattice with the space group Pbcm (no. 57) of the TFMBI and DFMBI crystals is lowered to the monoclinic lattice with the symmetric space group P 2 1 / c (no. 14). In contrast, antiferroelectric TCMBI is a polar crystal ( Fig. 1e ); the pseudo-orthorhombic symmetry of the polar space group Pmc 2 1 (no. 26) is lowered to that of the P 2 1 (no. 4) monoclinic lattice. The dipole moment component along the transverse molecular axes is arranged in an antiparallel manner, causing antiferroelectricity along the crystal a -axis, whereas that along the longitudinal axes cannot be cancelled out by the crystal symmetry, and permanent polarity is retained along the b direction normal to the hydrogen-bonded chains. Thermal properties For all five compounds, the temperature-dependent permittivity measured along the dipolar chains simply increases with temperature at least up to ~360–380 K ( Supplementary Figs S2 and S4 and Supplementary Discussion ) without any peak anomaly indicative of the Curie point. Thus, the ferroelectric or antiferroelectric phase persists from room temperature to far above room temperature. These compounds, except DC-MBI, did not display any phase transitions in differential scanning calorimetry (DSC) measurements until the samples gradually start to sublime at around 400–420 K. For DC-MBI, we found a first-order phase transition with a large hysteresis at high temperature; exothermic and endothermic peaks appeared at 369 and 399 K, respectively ( Supplementary Fig. S4a ). The discovery of ferroelectricity provides firm evidence for proton tautomerism, which comprises proton transfer and concomitant π-bond switching. This intriguing issue has long been studied in both the solution and solid states and also been addressed in relation to the large permittivity observed along the hydrogen-bonded chains of imidazole-related compounds [21] . The ac electric fields employed for the permittivity measurements are a few orders of magnitude smaller than that required for polarization reversal, and thus can probe only local fluctuations of the proton tautomerism and/or the bound motion of charged kink solitons on the hydrogen-bonded chains. As demonstrated for some benzimidazoles, this response may be tiny or even silent, regardless of the ferroelectricity or antiferroelectricity, especially when the Curie temperature is far above room temperature. In contrast, the reversal of a large polarization manifests collective switching that occurs in the whole crystal under a sufficiently large electric field. Incidentally, we note that in previous studies on the ferroelectricity of some imidazolium salts with inorganic anions [22] , [23] , it was reported that the ferroelectricity arises from the orientational order–disorder phenomena of both dipolar component ions, whereas completely protonated imidazolium cations cannot trigger collective proton dynamics. In addition to the chemical and thermal stability, the imidazole moieties have some advantages in terms of their substituent diversity. We found that the linear hydrogen-bonded chains can be aligned in various three-dimensional architectures. This feature is quite promising for finding new paradigms with various structure–property relationships, for instance, such as crystal symmetry and dimensionality. Polarity switching over two dimensions as seen for MBI is significantly advantageous for improving the polarization performance of the randomly orientated polycrystalline state, such as the thin-film form, compared with the uniaxial polarity available in other organic ferroelectrics except TEMPO [24] (tanane). An improved crystal symmetry also permits the formation of non-180° domains (that is, the 90° domain for MBI), which have often been utilized as high-performance ferroelectric or piezoelectric properties in ferroelectric oxides. These features suggest that there is a possibility of uniquely engineering the ferroelectric domains for organic electronic and optoelectric devices. The observation of both ferroelectricity and antiferroelectricity in the imidazole sequence can be related to the minute energy difference between their polar and antipolar arrangements. These findings recall the excellent electromechanical response in some piezoelectric lead zirconate titanate systems achieved by the electric-field-induced antiferroelectric to ferroelectric phase transition. It should also be noted that many imidazole-related compounds with various substituents are available from commercial sources and well-established chemical synthesis, and ferroelectric MBI is sold at low prices. Preparation and calorimetry All the purchased benzimidazoles were purified by recrystallization from alcohol (methanol, ethanol or 2-propanol) and/or temperature-gradient sublimation in vacuum until the coloured impurities were completely eliminated. Single crystals of MBI, DC-MBI and DFMBI were prepared by vacuum sublimation, whereas single crystals of TFMBI and TCMBI were grown by slow evaporation of the ethanol and 2-propanol solutions, respectively. The thermal properties were examined using a differential scanning calorimeter (SII DSC6100) with the temperature calibration performed using the melting point of indium (429.8 K). The sample was encapsulated in an aluminium pan and heated at a rate of 5 K min −1 . Electric measurements All the electric measurements were taken from single crystals with gold-paste electrodes. The dielectric permittivity was obtained by measuring the capacitance with an LCR metre. The P–E hysteresis curves were collected on a ferroelectrics evaluation system (Toyo Corporation, FCE-1) consisting of a current/charge–voltage converter (Toyo Corporation Model 6252), an arbitrary waveform generator (Biomation 2414B), an analogue-to-digital converter (WaveBook 516) and a voltage amplifier (NF Corporation, HVA4321). Both the dielectric hysteresis measurements and the modified double-wave method measurements were performed with a high-voltage triangular wave field and various alternating frequencies. The benzimidazole crystals were immersed in silicone oil to avoid electric discharge; the maximum electric field exceeded 30 kV cm −1 . High-temperature dielectric hysteresis measurements were conducted by heating the sample in the oil bath. X-ray crystallographic analysis The X-ray intensity data were collected on a Rigaku AFC7R four-circle diffractometer equipped with a Mercury CCD (charge-coupled device) area detector (graphite-monochromatized MoKα radiation) for the DFMBI and DC-MBI crystals at room temperature. For the MBI, TCMBI and TFMBI crystals, the measurements at room temperatures were performed on a Rigaku DSC imaging plate system using Si-monochromatized synchrotron radiation ( λ =0.9995 or 0.6878 Å) at the BL-8 A beamline of the Photon Factory, High Energy Accelerator Research Organization (KEK). All the calculations were performed using the CrystalClear, Rapid-AUTO and CrystalStructure crystallographic software packages of Molecular Structure Corporation and Rigaku Corporation. For the compounds investigated here, automatic symmetric analysis suggested a higher symmetry because symmetry lowering originates mainly from the locations of protons. The choice of a lowered symmetry gave chemically reasonable structures and was further justified by the present observations of ferroelectricity or antiferroelectricity. The final refinements were undertaken with anisotropic atomic displacement parameters for the non-hydrogen atoms and with isotropic parameters for the hydrogen atoms, except for those calculated on the aromatic moieties. CCDC-909439-909443 contains the supplementary crystallographic data for this paper. These data can be obtained free of charge from the Cambridge Crystallographic Data Centre via www.ccdc.cam.ac.uk/data_request/cif . PFM measurements The PFM measurements were carried out using a commercially available scanning probe microscope (Asylum MFP-3D) with a Ti/Ir-coated Si tip (Asylum Research). To achieve a good signal-to-noise ratio, we performed in-plane PFM measurements at 807 kHz, which is close to a torsional contact resonance frequency of the cantilever (~835 kHz). For imaging, an ac voltage of 1.3 V peak-to-peak was applied. To identify the direction of local polarization P local in the MBI crystal, in-plane PFM images were collected under different cantilever geometries ( Supplementary Fig. S6 ). How to cite this article: Horiuchi, S. et al . Above-room-temperature ferroelectricity and antiferroelectricity in benzimidazoles. Nat. Commun. 3:1308 doi: 10.1038/ncomms2322 (2012).